Outlines of the pore in open and closed conformations describe the gating mechanism of ASIC1 The proton-activated sodium channel ASIC1 belongs to the ENaC/Degenerins family of ion channels. Little is known about gating of the pore in any member of this class. Here we outline the shape of the ion pathway of ASIC1 in the open and closed conformations by measuring apparent rates of cysteine modification by thiol-specific reagents in the two transmembrane helices that form the pore (TM1 and TM2). Closed channels have a narrowing in the external end of the pore, whereas open channels have a narrowing midway, the length of TM2 that serves as selectivity filter. Thus, gating of the pore entails straightening the tilt of TM2 without significant rotation. The findings imply that the external narrowing serves as opening, closing and desensitization gate, and that the selectivity filter of ASIC1 is a transient structure that assembles in the open state and is pulled apart in the closed state. ASIC1 is a proton-activated sodium channel found in the plasma membrane of most neurons of the mammalian nervous system where it modulates synaptic transmission, induction of fear and memory, and nociception in peripheral neurons [1] , [2] . Structurally, ASIC1 is a trimer of identical or homologous subunits. Each subunit has two transmembrane segments (TM1 and TM2), short intracellular amino- and carboxy-termini, and a large extracellular domain. This architecture is the hallmark of all members of the ENaC/Degenerins family regardless of their particular function and mode of activation. Gouaux and his group have solved two atomic structures of chicken ASIC1 both in shut non-conducting conformations [3] , [4] . These structures correspond most likely to desensitized states of the channel, as the crystallization trials in both instances were conducted at low pH. Whereas the extracellular domain of the channel superimposes in these structures, the architecture of the transmembrane helices is markedly different. In the first version, which corresponds to a channel with truncated N- and C-termini, the ion pathway is collapsed [3] , whereas in the second version, which includes most of the N- and C-termini, crossing of the three TM2s occludes the external access to the pore [4] . Beyond the occlusion, the transmembrane segments separate to form a wide inner vestibule ( Fig. 1a ). The carbonyl of Gly-432 and the carboxylic group of Asp-433 in TM2 form the external side of the occlusion and also coordinate a Cs + ion suggesting that those two residues form a structure that functions as the desensitization gate and as the selectivity filter. 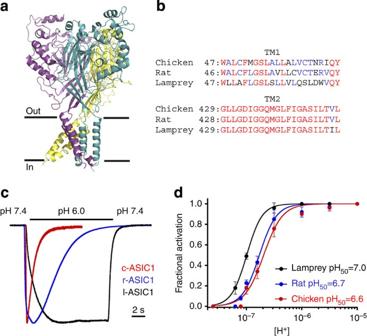Figure 1: Comparison of lamprey ASIC1-C74H with chicken and rat ASIC1. (a) Crystal structure of chicken ASIC1 viewed parallel to the membrane plane. Each subunit of the trimer is shown in ribbon representation of a different colour. The horizontal lines demarcate the limits of the plasma membrane enclosing the transmembrane helices (TM1 and TM2) of the subunits. Out, external; In, internal. (b) Amino-acid alignment of TM1 and TM2 of chicken, human and lamprey ASIC1. Identical residues are in red, conserved in blue, and different in black. (c) Time-course of normalized whole-cell currents of rat, chicken and lamprey-C74H evoked by changing the external pH from 7.4 to 6.0. Bar below traces indicates the time scale. Membrane potential was held at −60 mV and 120 mM Na+was the conducting cation in the bath. (d) Concentration–response relationships for H+of rat, chicken and lamprey-C74H ASIC1. Data points are the mean±standard deviation of at least 4 cells. Lines are the fit of the data to equation (1), pH50=−logEC50. Figure 1: Comparison of lamprey ASIC1-C74H with chicken and rat ASIC1. ( a ) Crystal structure of chicken ASIC1 viewed parallel to the membrane plane. Each subunit of the trimer is shown in ribbon representation of a different colour. The horizontal lines demarcate the limits of the plasma membrane enclosing the transmembrane helices (TM1 and TM2) of the subunits. Out, external; In, internal. ( b ) Amino-acid alignment of TM1 and TM2 of chicken, human and lamprey ASIC1. Identical residues are in red, conserved in blue, and different in black. ( c ) Time-course of normalized whole-cell currents of rat, chicken and lamprey-C74H evoked by changing the external pH from 7.4 to 6.0. Bar below traces indicates the time scale. Membrane potential was held at −60 mV and 120 mM Na + was the conducting cation in the bath. ( d ) Concentration–response relationships for H + of rat, chicken and lamprey-C74H ASIC1. Data points are the mean±standard deviation of at least 4 cells. Lines are the fit of the data to equation (1), pH 50 =−logEC 50 . Full size image Though the atomic structures of ASIC1 confirmed the subunit stoichiometry of the channel and provided detailed information of the conformation of the extracellular domain, fundamental questions of the architecture of the ion pathway and how the transmembrane helices arrange in the open and closed states of the pore remain unanswered. Towards this end, we have conducted cysteine-scanning mutagenesis of TM1 and TM2 and modification by thiol reagents [5] together with patch clamp analysis on ASIC1. The pattern and speed of reaction of cysteines with thiol-specific reagents outlined different shapes of the ion pathway in the open and closed conformations and identified the positions of the closing gate and the selectivity filter. Together, the results allow the proton-evoked gating movements of the transmembrane helices of ASIC1 to be inferred. ASIC1 channel Experiments were conducted on lamprey ASIC1 (lASIC1) that shares almost identical sequence of TM2 with chicken and human ASIC1 ( Fig. 1b ) [6] , but most importantly because lASIC1 exhibits distinct properties that made possible to implement the experimental approach used in this work. First, the low desensitization rate of lASIC1 keeps channels open over long exposures to external protons ( Fig. 1c ). Second, as the reaction of cysteine with thiol-specific reagents slows down as the pH decreases, it was crucial to use a channel with high affinity to protons, lASIC1 half-maximal activation is pH 50 7.0 ( Fig. 1d ) [7] . Finally, contrary to chicken and mammalian ASIC1, which are rendered non-functional by cysteine substitutions of most residues in TM2, lASIC1 is quite tolerant to mutagenesis. Furthermore, lASIC1 does not have cysteines in the transmembrane helices, and the only cysteine in the extracellular domain that is not engaged in the formation of a disulfide bond, Cys-74, was substituted by His to mimic human ASIC1. Cysteine scanning of TM2 and modification by MTS reagents The goal was to identify the narrowest segments of the ion pathway in the open and in the closed conformations. To that end, we used accessibility of cysteines to modification by methanethiosulfonate reagents (MTS) applied from the external or the internal side of the channel in either the open (outside pH 6.8) or the closed state (outside pH 7.4). We first substituted each amino acid in lASIC1 TM2 from Gly-429 to Leu-450 by cysteine residues. Of the 22 mutations, 12 produced non-functional channels when currents were elicited by external solutions in the pH range of 7.0 to 5.0. A 10 min pre-treatment with various metal chelating/reducing agents, such as 3 mM dithiothreitol, 0.1 mM 2,3-dimercaptopropanesulfonate 0.1 mM bis-2-mercaptoethylsulfone and 1.0 mm tris(2-carboxyethyl)phosphine hydrochloride, to reduce spontaneous disulfide bond formation and remove divalent cations, were ineffective in restoring function to the mutants. Thus, intersubunit disulfide bonds or creation of high-affinity binding sites for divalent cations (Cd 2+ and Ni 2+ ) are unlikely explanations for the suppression of current in the mutants. To extend the number of positions amenable to testing, we constructed trimers of three subunits linked head to tail and inserted the mutation into only one of the three subunits. 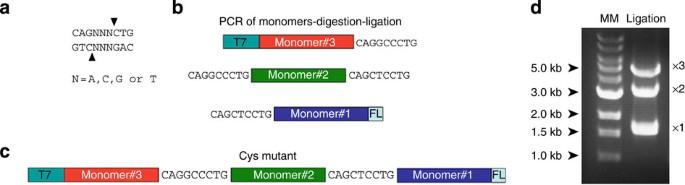Figure 2:In vitromethod for the construction of trimers. (a) DNA recognition sequence of AlwNI restriction enzyme, where N is any nucleotide. (b) Cartoon of PCR products of monomers #1, #2, and #3. Different complementary sequences attached to the ends of the monomers ensure that the ligation reaction proceeds only in the correct order and orientation of the three monomers. (c) Final ligation product of three monomers in the correct order with monomer#2 carrying the Cys mutation and monomer#3 the Flag epitope at the carboxy terminus (FL). (d) Products of a ligation reaction resolved in an agarose gel and stained with ethidium bromide. The three bands correspond to monomers (x1), dimers (x2) and trimers (x3). MM=1 Kb DNA molecular marker. The final product was used as template for synthesis of cRNA using T7 RNA polymerase. Owing to intractable recombination in Escherichia coli , we designed a method to make the trimers in vitro as described in methods and Figure 2 . Expression of trimers with a single mutated protomer rescued function in three positions, though the level of current was a fraction ≤0.3 of wild-type channels. Only one position, G443, produced enough current to conduct experiments in excised patches. Abundance of surface channels was analysed by western blots of biotinylated intact cells. Functional and non-functional mutants yielded similar levels of expression indicating that the absence of proton-evoked currents could not be explained by defects in synthesis/traffic of mutant channels but rather by functional defects induced by the mutations ( Supplementary Fig. S1 ). Figure 2: In vitro method for the construction of trimers. ( a ) DNA recognition sequence of AlwNI restriction enzyme, where N is any nucleotide. ( b ) Cartoon of PCR products of monomers #1, #2, and #3. Different complementary sequences attached to the ends of the monomers ensure that the ligation reaction proceeds only in the correct order and orientation of the three monomers. ( c ) Final ligation product of three monomers in the correct order with monomer#2 carrying the Cys mutation and monomer#3 the Flag epitope at the carboxy terminus (FL). ( d ) Products of a ligation reaction resolved in an agarose gel and stained with ethidium bromide. The three bands correspond to monomers (x1), dimers (x2) and trimers (x3). MM=1 Kb DNA molecular marker. The final product was used as template for synthesis of cRNA using T7 RNA polymerase. Full size image Initially, we used MTSET (diameter ~5.8 Å), which is a membrane-impermeable reagent, but only residues located in the amino- or carboxy-end of TM1 and TM2 reacted with this compound. Switching to MTSEA (diameter ~3.6 Å), a smaller but membrane-permeable MTS compound [8] , increased the number of reactive positions. All subsequent experiments were then conducted with MTSEA. 15 mM of free cysteine was added to the trans side of MTSEA to quench the reagent crossing the membrane, unless indicated otherwise. In addition, as MTSEA releases protons by spontaneous hydrolysis (half-life ~12 min at pH 7.0 and 20 °C) [7] , solutions with MTS reagents contained buffer (Hepes or MES) in concentrations predicted by the Henderson–Hasselbach equation to keep the pH from changing by ≤0.1 pH units. Mean values of the reaction rates were obtained for each functional substitution in TM2. 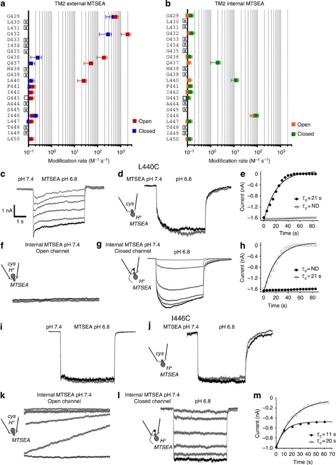Figure 3: Modification rates of cysteine substitutions in TM2 induced by MTSEA. Applied from (a) the external side of the channel in the open (red) or closed (blue) conformations, and from (b) the internal side of the channel in the open (orange) or in the closed (green) conformations. Each data point is the mean±s.d. of 4 experiments. White squares indicate rescued channel function by a trimer expressing the mutation in a single subunit. Crossed squares indicate non-functional channels. (c) Representative example of currents from an outside-out patch expressing L440C modified by external application of MTSEA to open channels, pH 6.8. Each current trace represents a sweep of 5 s at pH 7.4 and 5 s at pH 6.8. The first trace is the control without MTSEA and is shown in black; subsequent sweeps after addition of MTSEA are in gray. (d) Outside-out patch with externally applied MTSEA in the closed state, pH 7.4. (e) Graph of the time courses of experiments shown in (c) and (d). (f) Inside-out patch with MTSEA applied to the internal side of channels in the open state (pipette solution pH 6.8). (g) Inhibition of currents by internal MTSEA crossing the membrane while the channel is closed. Free cysteine was omitted from the pipette solution. (h) Graph of the time courses of experiments shown in (f) and (g). (i) Outside-out patch expressing I440C exposed to MTSEA in the open state. Only the control current (black) and the last (gray) sweep out of 15 containing MTSEA are shown. (j) Outside-out patch exposed to MTSEA in the closed state. First and last sweeps of the experiment are shown. (k) Outside-out patch: open channels exposed to internal MTSEA. (l) Outside-out patch: MTSEA modification of closed channels from the internal side. MTSEA reaches I446 by crossing the membrane, free cysteine was omitted from the pipette solution. (m) Graph of the time courses of experiments shown in (k) and (l). Membrane potential was −60 mV. Time and amplitude scales are the same for all examples. Cartoons illustrate the configuration of the corresponding patch experiment and the side of H+, MTSEA, and cysteine applications. Figure 3a shows the reaction rates measured in the open (red) and closed (blue) conformations, when MTSEA was applied to the external side of the pore whereas Figure 3b shows corresponding rates (open in orange, closed in green), when the reagent was applied from the internal side of the pore. These results indicate that in the closed state, the channel presents a barrier that prevents passage of external MTSEA past the outer segment of TM2 (G432). In the open state, the pore widens and lets MTSEA reach down to residue L440 that is located in the middle of TM2. In contrast, internally applied MTSEA reaches the midpoint of TM2 (Q437 and L440) in the closed state but reaches only the distal segment of TM2 (I446) in the open state. Figure 3: Modification rates of cysteine substitutions in TM2 induced by MTSEA. Applied from ( a ) the external side of the channel in the open (red) or closed (blue) conformations, and from ( b ) the internal side of the channel in the open (orange) or in the closed (green) conformations. Each data point is the mean±s.d. of 4 experiments. White squares indicate rescued channel function by a trimer expressing the mutation in a single subunit. Crossed squares indicate non-functional channels. ( c ) Representative example of currents from an outside-out patch expressing L440C modified by external application of MTSEA to open channels, pH 6.8. Each current trace represents a sweep of 5 s at pH 7.4 and 5 s at pH 6.8. The first trace is the control without MTSEA and is shown in black; subsequent sweeps after addition of MTSEA are in gray. ( d ) Outside-out patch with externally applied MTSEA in the closed state, pH 7.4. ( e ) Graph of the time courses of experiments shown in ( c ) and ( d ). ( f ) Inside-out patch with MTSEA applied to the internal side of channels in the open state (pipette solution pH 6.8). ( g ) Inhibition of currents by internal MTSEA crossing the membrane while the channel is closed. Free cysteine was omitted from the pipette solution. ( h ) Graph of the time courses of experiments shown in ( f ) and ( g ). ( i ) Outside-out patch expressing I440C exposed to MTSEA in the open state. Only the control current (black) and the last (gray) sweep out of 15 containing MTSEA are shown. ( j ) Outside-out patch exposed to MTSEA in the closed state. First and last sweeps of the experiment are shown. ( k ) Outside-out patch: open channels exposed to internal MTSEA. ( l ) Outside-out patch: MTSEA modification of closed channels from the internal side. MTSEA reaches I446 by crossing the membrane, free cysteine was omitted from the pipette solution. ( m ) Graph of the time courses of experiments shown in ( k ) and ( l ). Membrane potential was −60 mV. Time and amplitude scales are the same for all examples. Cartoons illustrate the configuration of the corresponding patch experiment and the side of H + , MTSEA, and cysteine applications. Full size image Representative examples of two relevant mutants: L440C and I446C are shown in Figure 3c–m . The first current trace, before MTSEA application is marked in black, whereas sweeps that followed MTSEA application are marked in grey. For clarity, some examples show only the first and last sweeps of the experiment. The drawing adjacent to the current traces depicts the configuration of the patch (inside-out or outside-out), the composition of the internal and external solutions, and the side of MTSEA reactivity relative to the pore. Because we had access to fast solution exchange only from one side of the membrane, in some experiments, free cysteine was removed from the pipette solution to let MTSEA react from the trans side ( Fig. 3g,l ). The protocol described in Figrue 3g was also conducted with cysteine in the external solution (pH 6.8) to ensure back diffusion of MTSEA from the pipette to the bath was quenched and rapidly removed by the perfusion system ( Supplementary Fig. S2 ). Representative examples of MTSEA modification of other positions in TM2 are shown in Supplementary Figure S3 . Cysteine scanning of TM1 and modification by MTS reagents Following the approach described above, we substituted each position in TM1 from Trp-47 to Tyr-68 by cysteine residues. Of the 22 mutants, 2 were non-functional (F51C and W47C) and were not rescued by trimers carrying a single mutated subunit. The patterns of reactivity to external ( Fig. 4a ) and internal ( Fig. 4b ) applications in the open and closed states were assessed following the techniques described for TM2. The only mutant in TM1 that changed by MTSEA treatment was W65C. As we have previously described, substitutions of position W65 induce desensitization to lamprey ASIC1 [6] ; thus, channels with the mutation W65C exhibit a transient peak and a slowly desensitizing component ( Fig. 4c,d ). 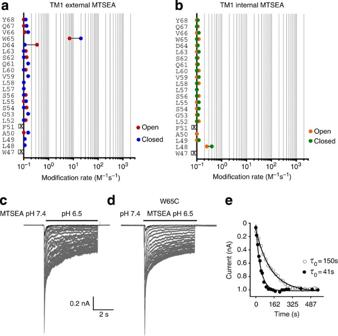Figure 4: Modification rates of cysteine substitutions in TM1 by MTSEA. applied from the (a) external side of the channel pore in the open (red squares) or closed (blue squares) conformations. (b) Modification rates of MTSEA applied from inside the channel in the open (orange) and closed (green) conformations. Each data point is the mean±s.d. of 4 experiments. (c) Outside-out patch expressing the mutant W65C. MTSEA was applied to the external side of closed channels, pH 7.4. (d) Outside-out patch with MTSEA applied to the external side of open channels, pH 6.5. (e) Time-course of peak currents from experiments shown incandd,τoandτcare open and closed time constants. Membrane potential −60 mV. Time and amplitude scales are the same incandd. MTSEA increased the magnitude of both components; Figure 4e shows the time course of the peak current in the open and closed states. Residue W65C was equally modified by external MTSEA and MTSET, indicating that the entrance of the pore is wider than the rest of the ion pathway in both open and closed conformations. Additionally, as residues in TM1 are not exposed to water in either closed or open conformations, with exception of the external segment that bears W65, it appears that most of TM1 does not line the ion pathway. Figure 4: Modification rates of cysteine substitutions in TM1 by MTSEA. applied from the ( a ) external side of the channel pore in the open (red squares) or closed (blue squares) conformations. ( b ) Modification rates of MTSEA applied from inside the channel in the open (orange) and closed (green) conformations. Each data point is the mean±s.d. of 4 experiments. ( c ) Outside-out patch expressing the mutant W65C. MTSEA was applied to the external side of closed channels, pH 7.4. ( d ) Outside-out patch with MTSEA applied to the external side of open channels, pH 6.5. ( e ) Time-course of peak currents from experiments shown in c and d , τ o and τ c are open and closed time constants. Membrane potential −60 mV. Time and amplitude scales are the same in c and d . Full size image Changes in ion selectivity and conductance produced by G443C The previous results indicate that G443 is located in the narrowest segment of the ion pathway in the open state. This observation qualifies G443 as the potential site for the selectivity filter. Consistent with this notion is the high degree of conservation of the sequence G443–A444–S445 in all ASICs known to date. In addition, the function of lASIC1 was highly sensitive to minor perturbations of the sequence encoded by those three residues. All substitutions tested (C, A, S, I, L, V, Q, E, K) abolished currents in rat and lamprey ASIC1. However, function was preserved, when the mutation G443C was present in only one of the three subunits of lASIC1 (trimer-G443Cx1). Those channels expressed currents with the same proton affinity as wild-type, although the total current magnitude was reduced by 65%. Changes in reversal potential in the presence of Na + , K + , Li + or Cs + were used to calculate permeability ratios. The permeability ratios of the trimer-G443Cx1 were P Na /P Li :3, P Na /P K :5.8, P Na /P Cs :12, whereas of wild-type channels examined under identical conditions the values were P Na /P Li :1.4, P Na /P K :5, P Na /P Cs :28 ( Fig. 5a,d ). The unitary chord conductance (voltage range −60 to + 60 mV) measured in the presence of 120 mM external Na + and nominal zero Ca 2+ was 28±5 and 42±4 pS for the mutant and wild type, respectively ( Fig. 5b,e ). Unitary current amplitudes estimated from all-points histograms were 0.44 and 1.32 pA measured at a membrane potential of −60 mV ( Fig. 5c,f ). Together, these results are consistent with G443 being part of the selectivity filter. 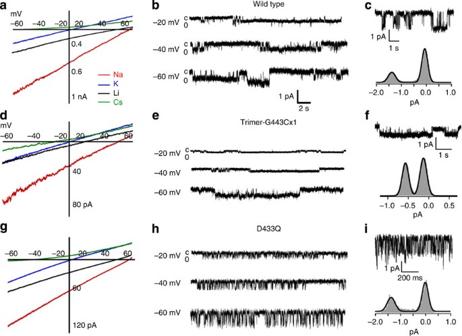Figure 5: Ion selectivity and conductance of wild type and mutants. (a) IV-curves of wild-type lASIC1 in the presence of 120 mM K+in the pipette and 120 mM Na+, Li+, K+or Cs+in the external solution, pH 6.8. (b) Representative traces of an outside-out patch containing a single channel activated by pH 6.8 at the indicated voltages. C, closed; O, open. (c) All point histogram of current amplitude recorded at −60 mV, 120 mM Na+and 1.5 mM Ca2+in the external solution. (d–f) Similar experiments conducted with a concatameric trimer (Trimer-G443Cx1) that has the mutation G433C in only one monomer whereas the two other monomers are wild type. (g–i) Representative experiments of lASIC1-D433Q, the mutation is present in the three subunits of the trimer. Figure 5: Ion selectivity and conductance of wild type and mutants. ( a ) IV-curves of wild-type lASIC1 in the presence of 120 mM K + in the pipette and 120 mM Na + , Li + , K + or Cs + in the external solution, pH 6.8. ( b ) Representative traces of an outside-out patch containing a single channel activated by pH 6.8 at the indicated voltages. C, closed; O, open. ( c ) All point histogram of current amplitude recorded at −60 mV, 120 mM Na + and 1.5 mM Ca 2+ in the external solution. ( d – f ) Similar experiments conducted with a concatameric trimer (Trimer-G443Cx1) that has the mutation G433C in only one monomer whereas the two other monomers are wild type. ( g – i ) Representative experiments of lASIC1-D433Q, the mutation is present in the three subunits of the trimer. Full size image Functional effects of mutants in the external narrowing Whereas G443 lies in the narrowest segment of the ion pathway in the open conformation, G432 and D433 are located in the external narrowing of the closed conformation. Channels bearing the mutation D433C in three or in a single subunit of lASIC1 were not functional; however, substitution by Gln in all three subunits produced functional channels with ion permeabilities P Na /P Li :1.6, P Na /P K :6.8, P Na /P Cs :30 ( Fig. 5g ), conductance 40±5 pS, and unitary amplitude 1.36 pA ( Fig. 5i ), which are not different from wild type. The kinetics of the mutant D433Q were however different from wild type; rather than long opening events of several seconds duration ( Fig. 5b,e ), D433Q had series of brief open and shut events that produced a flickering pattern ( Fig. 5e ) [9] . These results strengthen the notion that D433 is part of the constriction that serves as the gate in the closed conformation whereas G443 is in a constriction that serves as the selectivity filter in the open conformation. This study examines the outline of ASIC1 pore in the open and closed conformations using modification rates of cysteines in the transmembrane segments by thiol-specific reagents. The results indicate that only the external end of TM1 and most of TM2 are exposed to the pore lumen in the open and closed states. All the reactive positions in TM2 face the same side of the α-helix, suggesting that there is little rotation of TM2 in the transition from close to open. We found evidence that the diameter of ASIC1's ion pathway is narrow as most residues, with the exception of the ones located at the external and internal ends of TM1 and TM2, reacted only with MTSEA but not with MTSET. The apparent reaction rates of many positions were relatively slow. Two factors may have contributed: first, the relative high proton concentration (pH 6.8), used to examine the open states reduced the fraction of the reactive moiety (ionized-S − groups in cysteines) and thus slowed the reactions. Second, the overall small diameter of the ion pathway probably retarded the 'on-rate' of MTSEA reaction, in particular, with residues located deep in the pore. The pattern of reactivity of residues in the open state was different from that in the closed state. Accessibility of residues of lASIC1 in the open state was consistent with a constriction located midway of TM2, residues G443–A444–S445, whereas accessibility in the closed state was consistent with the presence of a narrowing in the outer segment, residues G432-D433. Features of residues in these two narrow segments are a high degree of conservation among all ASICs cloned to date and very low tolerance to mutagenesis; both observations underscore the functional importance of the identified segments. Mutations in the narrow segment of the open state indicate that it functions as the selectivity filter. This result agrees with previous mutagenesis studies conducted on ENaC, a channel closely related to ASIC1. The corresponding residues: αEnaC–G 587 , βEnaC–G 529 and γEnaC–S 541 change the permeability ratio of Na + and Li + and decrease the unitary conductance of ENaC [10] . In contrast, the narrow segment of the closed state (G432–D433) maps to the constriction assigned in the crystal structure as the desensitization gate, thus, the same structural element serves to shut the pore in the closed and in the desensitized states. An additional finding was that Cd 2+ (up to 50 μM) did not inhibit any of the functional mutants in lASIC1 (data not shown). This result contrasts to that obtained in the P2X receptor, which is also a trimer with each subunit formed by two transmembrane helices [11] . Cysteine scanning mutagenesis of rat P2X receptor produced high affinity Cd 2+ -binding sites (EC 50 ~2–20 μM) in three positions of TM2: T336C, V343C, and S345C (refs 12 , 13 ), which correspond to residues G436, G443 and S445 in ASIC1. A possible explanation for the resistance to Cd 2+ block is that the ion pathway of ASIC1 is narrower than the hydrated diameter of a Cd 2+ ion (8.52 Å) [14] . The open pore seems to be widest at the external entrance where it accommodates MTSET. As it traverses the membrane, the pore tapers down accommodating only MTSEA, and, at the level of the constriction formed by G443, it does not allow neither reagent. In contrast, in the P2X receptor, Cd 2+ enters deep into the pore and reaches the position corresponding to the narrow segment of ASIC1. Tolerance to mutagenesis and coordination of Cd 2+ at this site are signs that the P2X receptor has a wider pore than ASIC1. This also agrees with P2X receptor permeation by large organic cations, including guanidinium [15] . The observation that MTSEA passes beyond the segment G443–A444–S445 when applied from inside the closed channel indicates that the pore diameter at this level is wider in the closed than in the open conformation. The crystal structure shows these three residues as a slightly unwinding α-helix turn of TM2 lining an inner vestibule ( Fig. 6a ). Seen from inside, the carbonyl groups of G443 form the corners of an equilateral triangle with sides ~10.67 Å (dotted lines in Fig. 6b ). In contrast, our functional studies indicate that this part of the ion pathway is inaccessible by MTSEA in the open conformation. The inevitable implication of these observations is that the transition from closed to open entails a narrowing of the lumen of the inner vestibule that brings together the TM2 segments and reduces the dimensions of the inner vestibule to a diameter smaller than that of a Cs + ion (~3.3 Å). Therefore, the selectivity filter of ASIC1 is not a fixed structure, but it assembles when the channel opens and widens when the channel is closed/desensitized ( Fig. 6c,d ). Such a significant change in the geometry of the selectivity filter is an exception in the field of ion channels in particularly, because molecular sieving has been proposed as the basis for selecting Na + over K + in channels of the ENaC/Degenerins family [16] , [17] , [18] . It is unexpected that a channel that may rely on pore size to select the passing ions is also one that exhibits major changes in the diameter of the selectivity filter during gating. The notion that the selectivity filter of ion channels undergoes some degree of rearrangements during gating is not entirely foreign; analysis of the atomic structure together with detailed molecular dynamics free energy simulations have changed the classical snug-fit mechanism to more flexible binding sites influenced by local energetics (recently reviewed by Roux et al . [19] ). However, in those instances, the proposed structural changes are slight compared with the whole assembly of ASIC1 selectivity filter shown by our results. Because the crystal of ASIC1 in the shut conformation does not have an assembled functional selectivity filter, the structural basis for ion selectivity of ASIC1 remains still elusive. Whether only the carbonyl groups of the polypeptide backbone of G443–A444–S445, the side chain of A444 (the only residue in the triad facing the lumen), or perhaps all those elements coordinate passing ions remain open questions. The answer awaits resolution of the atomic structure of ASIC1 in the open conformation, which will provide the first molecular organization of a pore with a trimeric geometry that selects Na + over K + . 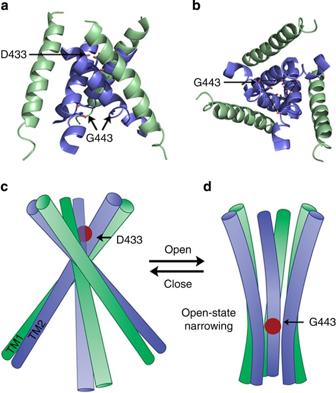Figure 6: Proposed rearrangement of TM1 and TM2 induced by H+. (a) Ribbon representation of the atomic structure of the transmembrane domain of chicken ASIC1 in the shut state viewed parallel to the membrane. TM1 is shown in green and TM2 in blue. Red sticks show residues D433 in the external constriction and G443 located in a stretched segment of the α-helix of TM2. (b) View from inside the pore. The carbonyl groups of G443 form an equilateral triangle (dashed lines) with sides of 10.7 Å. (c) and (d) Cartoons illustrating the predicted rearrangement of TM1 and TM2 evoked by proton activation. A decrease in the tilt of the transmembrane domains widens the external constriction and brings together the partially unfolded α-helix segments G433-A444-S445 to form a narrowing deeper in the pore that allows the passage of Na+ions (red dot) but not of larger molecules such as MTSEA. Figure 6: Proposed rearrangement of TM1 and TM2 induced by H + . ( a ) Ribbon representation of the atomic structure of the transmembrane domain of chicken ASIC1 in the shut state viewed parallel to the membrane. TM1 is shown in green and TM2 in blue. Red sticks show residues D433 in the external constriction and G443 located in a stretched segment of the α-helix of TM2. ( b ) View from inside the pore. The carbonyl groups of G443 form an equilateral triangle (dashed lines) with sides of 10.7 Å. ( c ) and ( d ) Cartoons illustrating the predicted rearrangement of TM1 and TM2 evoked by proton activation. A decrease in the tilt of the transmembrane domains widens the external constriction and brings together the partially unfolded α-helix segments G433-A444-S445 to form a narrowing deeper in the pore that allows the passage of Na + ions (red dot) but not of larger molecules such as MTSEA. Full size image In summary, the gating mechanism of ASIC1 can be explained by the alternate formation of two constrictions along TM2. In the closed state, the pore has a constriction in the outer segment formed by residues G432 and D433 that serves as closing and desensitization gate. Straightening of the ~50° angle of TM2 transitions the pore to the open state by widening the entrance while producing a new narrowing in the middle of TM2 that serves as the selectivity filter. This mechanism is similar to that proposed by Li et al . for the P2X receptor [13] where binding of the agonist molecule ATP also lessens the angle of the transmembrane helices resulting in expansion of the gate region in the external pore and in narrowing of the inner pore. Thus, two different families of trimeric ligand-gated ion channels –ASIC and P2X-, without protein sequence homology but with similar structure of the transmembrane domain, seem to share a comparable mechanism of opening the pore. Molecular biology Cysteine mutations were introduced in the cDNA of lamprey ASIC1-FLAG in pCR2.1 vector using QuickChange (Agilent). All DNA products were sequenced to confirm the presence of the mutations. Plasmids were linearized with Hind III restriction enzyme and transcribed in vitro using the T7 mMESSAGE mMACHINE kit (Ambion). Xenopus laevis oocytes were injected with 5 ng of cRNA. Oocytes were prepared by standard procedures [20] from frog ovaries purchased from Nasco (Fort Atkinson). In vitro construction of ASIC1 trimers Each monomer was amplified with high fidelity Taq polymerase using forward and reverse primers containing complementary sequences of the restriction enzyme AlwN. The forward primer of monomer#3 contained the sequence of the T7 promoter. The reverse primer of monomer#1 contained the Flag epitope. Products of the three PCR reactions were digested with AlwNI, isolated and ligated: 0.4 μg μl −1 of each monomer, 4 units of T4 ligase in a final volume of 20 μl for incubated at 12 °C over night. The whole ligation reaction was loaded on an agarose gel and the upper band corresponding to the trimer was isolated and purified. Approximately 2 μg of the trimer DNA was used as template in a standard 20 μl reaction of cRNA synthesis using the mMESSAGE mMACHINE kit (Agilent) with T7 RNA polymerase, according to the manufacturer's instructions. Electrophysiology Patch clamp recordings were conducted in the outside-out or inside-out configurations. Patch pipettes were pulled from PG150T glass (Warner Instruments) to tip diameter of 2–4 μm after heat polishing. In outside-out patches, the pipette solution was (mM): 120 KCl, 5 EDTA, 20 HEPES titrated with KOH to pH 7.4, and 15 mM cysteine, unless indicated. In inside-out patches, the pipette solution was pH 6.8. Bath and activating solutions were (mM) 120 NaCl, 2 mM KCl, 1 mM CaCl 2 , and 40 HEPES buffered to pH 7.4 or 6.8. Activating or modifying solutions were applied using a Perfusion Fast Step device SF-77B (Warner Instruments) onto which were mounted six perfusion pipettes. The data acquisition program Pulse in turn controlled the SF-77B. Recordings were made using EPC-9 amplifier and the Pulse acquisition program (HEKA Electronic). Membrane potential was held at −60 mV, unless indicated. Experiments were conducted at room temperature. MTSEA or MTSET (Anatrace) were prepared fresh in 1 ml solutions of pH 7.4 or 6.8 and were replaced every 15 min. Data analysis Apparent proton affinity was calculated with where I is the normalized current at a give concentration of protons ([H + ]), EC 50 is the [H + ] producing half-maximal currents and n is the Hill coefficient. Permeability ratios of monovalent cations. Voltage ramps from 60 to −60 mV were applied over one second on outside-out patches perfused with solutions containing 120 mM of single monovalent cations: Na + , Li + , K + , or Cs + buffered at pH 6.8. Relative permeabilities were calculated according to where E rev A indicates the reversal potential for Na + , RT/zF has the usual meaning, and [ B ] o is the concentration of the ion in the external bath, 120 mM (ref. 21 ). Time constants for modification (τ) were obtained by fitting relaxations with a single exponential function, and apparent modification rates ( R ) were calculated according to where [ M ] is the concentration of MTSEA. How to cite this article: Li, T. et al . Outlines of the pore in open and closed conformations describe the gating mechanism of ASIC1. Nat. Commun. 2:399 doi: 10.1038/ncomms1409 (2011).